Structural and evolutionary versatility in protein complexes with uneven stoichiometry Proteins assemble into complexes with diverse quaternary structures. Although most heteromeric complexes of known structure have even stoichiometry, a significant minority have uneven stoichiometry—that is, differing numbers of each subunit type. To adopt this uneven stoichiometry, sequence-identical subunits must be asymmetric with respect to each other, forming different interactions within the complex. Here we first investigate the occurrence of uneven stoichiometry, demonstrating that it is common in vitro and is likely to be common in vivo . Next, we elucidate the structural determinants of uneven stoichiometry, identifying six different mechanisms by which it can be achieved. Finally, we study the frequency of uneven stoichiometry across evolution, observing a significant enrichment in bacteria compared with eukaryotes. We show that this arises due to a general increased tendency for bacterial proteins to self-assemble and form homomeric interactions, even within the context of a heteromeric complex. Interactions between proteins often result in their assembly into complexes with defined quaternary structure topologies. Given that protein complexes are essential to most biological processes, there is a clear need to understand the principles by which assembly occurs and quaternary structure is organized. Although proteomic analyses have provided tremendous insights into the subunit compositions of protein complexes [1] , [2] , [3] , most of the deep insight into protein complex assembly and quaternary structure has come from detailed structural investigations. We now have experimental data on the assembly, structure, dynamics and function of a wide range of protein complexes, ranging from small complexes such as haemoglobin [4] , [5] to large macromolecular machines such as the proteasome [6] , [7] , [8] . Furthermore, structure-based protein complex design has become feasible in certain cases [9] , [10] , [11] , [12] . Finally, structural bioinformatic approaches combined with mass spectrometry have revealed that most complexes assemble via ordered pathways that are generally conserved, and that show striking similarities to their evolutionary pathways [13] , [14] , [15] . Symmetry is a key feature of many protein complexes. Most homomeric complexes (that is, those containing only a single type of subunit) and many heteromeric complexes (that is, those with multiple distinct subunits) are symmetric and can be classified into a limited number of closed symmetry groups [16] , [17] , [18] , [19] . Despite this preponderance of symmetry in crystallized protein complexes, asymmetry is also common and often important [20] , [21] , [22] , [23] . Although many complexes can be classified into closed symmetry groups, there are often small-to-moderate conformational differences observed between sequence-identical subunits within the same ‘symmetric’ homomer [17] , [24] . Furthermore, any heteromer that has uneven subunit stoichiometry (that is, 2:1 or 3:1) will inherently have some degree of asymmetry. This is because, to assemble a complex with uneven stoichiometry, different subunits of the same type must necessarily exist in different local environments. This can be seen in Fig. 1 , where complexes with even and uneven stoichiometry are shown. For the complex with uneven 2:1 stoichiometry, the single low stoichiometry (L) subunit binds two high stoichiometry (H) subunits through different surfaces. As each H subunit interacts with a different region on the L subunit, they are in non-equivalent positions within the complex. 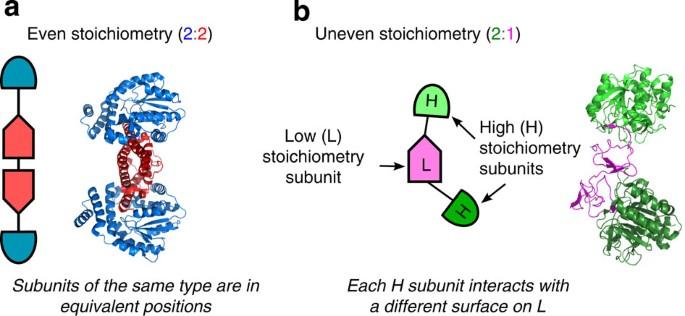Figure 1: Even versus uneven stoichiometry in heteromeric protein complexes. Examples of protein complexes with (a) even (Streptococcus pyogenesε/ζ complex; PDB ID: 1GVN) and (b) uneven (tomato inhibitor-II in complex with subtilisin Carlsberg; PDB ID: 1OYV) stoichiometry. Figure 1: Even versus uneven stoichiometry in heteromeric protein complexes. Examples of protein complexes with ( a ) even ( Streptococcus pyogenes ε/ζ complex; PDB ID: 1GVN) and ( b ) uneven (tomato inhibitor-II in complex with subtilisin Carlsberg; PDB ID: 1OYV) stoichiometry. Full size image Several well known complexes have uneven stoichiometry [25] , [26] , [27] . The mechanisms by which this asymmetric uneven stoichiometry can been formed have been discussed for some specific cases [28] , [29] . In general, however, little attention has been paid to the differences between complexes with even or uneven stoichiometry, and there has been no systematic analysis of the phenomenon. Here, we perform a detailed investigation into protein complexes with uneven stoichiometry. We find that uneven stoichiometry is common in heteromeric complexes and that there is likely to be a strong tendency for the uneven stoichiometry observed crystallographically to also be present in vivo . We then illustrate how uneven stoichiometry can be facilitated by diverse structural mechanisms. Finally, we consider the occurrence of uneven stoichiometry across evolution, observing a striking tendency for bacterial complexes to be enriched in uneven stoichiometry compared with eukaryotes. We show that this arises as part of a general increased propensity for bacterial proteins to form homomeric interactions. Uneven stoichiometry is common We start with a set of 1,832 non-redundant heteromeric crystal structures, of which 179 (9.8%) have uneven stoichiometry. If we consider only the 722 heteromers with at least one repeated subunit (that is, ignoring stoichiometries of 1:1, 1:1:1 and so on), then 24.8% have uneven stoichiometry. Next, we plot the percentages of complexes with uneven stoichiometry for heteromers with varying numbers of distinct subunit types ( Fig. 2a ). There is a strong tendency for uneven stoichiometry to increase in complexes with more subunit types. This makes physical sense: the more distinct subunit types there are within a complex, the greater potential there is for at least one to vary in stoichiometry. Importantly, this result also suggests that the frequency of uneven stoichiometry might be even higher in vivo , given that complexes within the cell are likely to generally have more distinct subunit types than those from crystal structures [30] , [31] . 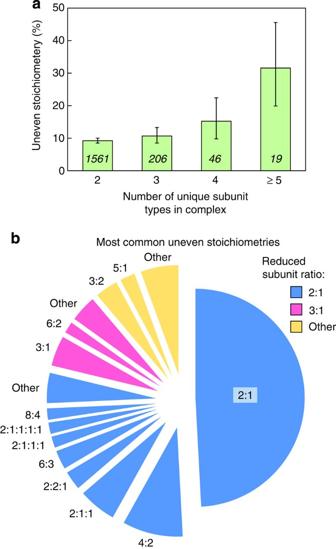Figure 2: Prevalence of protein complexes with uneven stoichiometry. (a) Percentage of heteromeric crystal structures with uneven stoichiometry, grouped by the number of unique subunit types (defined by sequence) in each complex. The numbers of heteromeric complexes (including both even and uneven stoichiometry) in each group are shown on the bars. Error bars represent 68% Clopper–Pearson binomial confidence intervals. (b) Pie chart showing the most common uneven stoichiometries in our data set. Stoichiometries are grouped by their reduced subunit ratio, which is the reduced ratio of H to L subunit repetitions (for example, stoichiometries of 4:2, 2:1:1 and 6:3 all have a subunit ratio of 2:1). Figure 2: Prevalence of protein complexes with uneven stoichiometry. ( a ) Percentage of heteromeric crystal structures with uneven stoichiometry, grouped by the number of unique subunit types (defined by sequence) in each complex. The numbers of heteromeric complexes (including both even and uneven stoichiometry) in each group are shown on the bars. Error bars represent 68% Clopper–Pearson binomial confidence intervals. ( b ) Pie chart showing the most common uneven stoichiometries in our data set. Stoichiometries are grouped by their reduced subunit ratio, which is the reduced ratio of H to L subunit repetitions (for example, stoichiometries of 4:2, 2:1:1 and 6:3 all have a subunit ratio of 2:1). Full size image We also utilized alternate sources of stoichiometry data. Of 182 non-redundant nuclear magnetic resonance (NMR) heteromers, 16 (8.8%) have uneven stoichiometries. Of 48 non-redundant electron microscopy (EM) heteromers, 14 (29.2%) have uneven stoichiometry. Finally, we used the IntAct Complex Portal [32] , which contains manually curated stoichiometry assignments based on direct physical interaction evidence using various experimental methods taken from the literature. After filtering for sequence redundancy and excluding those with structures in the PDB, 27 of the 176 (15.3%) heteromers have uneven stoichiometry. We plot the relationship between number of distinct subunit types and uneven stoichiometry for each of these data sets in Supplementary Fig. 1a . Figure 2b shows the most common uneven stoichiometries from our crystal structure data set. Nearly half of those complexes with uneven stoichiometry are 2:1 (49.2%). When considering complexes by their reduced subunit ratio (that is, the relative ratio of H subunit repetitions to L subunit repetitions), 78.8% are 2:1. Similar trends are observed for NMR, EM and IntAct complexes, although there are differences due to the much smaller data set sizes and the different types of complexes present in each ( Supplementary Fig. 1b ). Intracellular abundances reflect in vitro stoichiometry Many heteromers have uneven stoichiometry in vitro . Do these complexes also have uneven stoichiometry within the cell? Recent studies have demonstrated increased translational efficiency for the higher stoichiometry subunits within a complex [33] , [34] , suggesting that in vivo protein expression levels are often optimized for the same uneven stoichiometry observed in vitro . In another study, a high proportion of the pairwise interactions from complexes purified from human cells was estimated to have uneven stoichiometry, although such proteomic measurements are only approximate [3] . To investigate this further, we used PaxDB [35] to map intracellular protein abundance measurements from different organisms onto the subunits of uneven stoichiometry heteromers. For humans, we also utilized the tissue-specific abundance measurement available from the recent mass-spectrometry-based draft of the human proteome [36] . For each organism, we considered all pairs of subunits with uneven stoichiometry where abundance measurements were available for both subunits. In Fig. 3 , we plot the percentage of subunit pairs in which the H subunit is more abundant than the L subunit (green), versus the percentage of pairs where the L subunit is more abundant (pink). 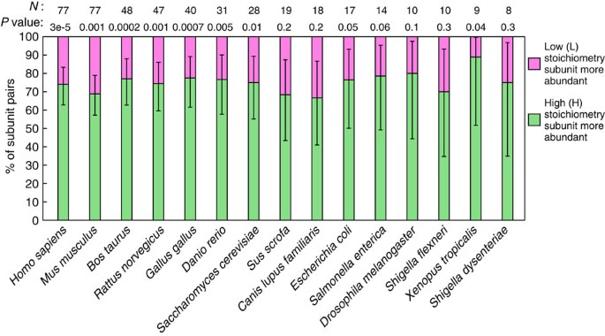Figure 3: Correspondence between subunit stoichiometry and intracellular abundance measurements. Non-redundant heteromeric pairs of subunits with different stoichiometries were mapped onto the protein-coding genes from different organisms for which intracellular abundance measurements are available in PaxDB, or Proteome DB for humans. For the tissue-specific measurements from Proteome DB, the median subunit ratio from different human tissues where measurements for both proteins are available was used. The percentage of pairs in which the higher stoichiometry subunit is more abundant (green) versus less abundant (pink) is plotted for each organism. The numbers of subunit pairs andPvalues (binomial test) are plotted above. For the PaxDB human measurements (not plotted here but included inSupplementary Data 4), H subunits were more abundant in 67/100 pairs (P=0.0009). Error bars represent 95% Clopper–Pearson binomial confidence intervals. Figure 3: Correspondence between subunit stoichiometry and intracellular abundance measurements. Non-redundant heteromeric pairs of subunits with different stoichiometries were mapped onto the protein-coding genes from different organisms for which intracellular abundance measurements are available in PaxDB, or Proteome DB for humans. For the tissue-specific measurements from Proteome DB, the median subunit ratio from different human tissues where measurements for both proteins are available was used. The percentage of pairs in which the higher stoichiometry subunit is more abundant (green) versus less abundant (pink) is plotted for each organism. The numbers of subunit pairs and P values (binomial test) are plotted above. For the PaxDB human measurements (not plotted here but included in Supplementary Data 4 ), H subunits were more abundant in 67/100 pairs ( P =0.0009). Error bars represent 95% Clopper–Pearson binomial confidence intervals. Full size image There is a strong tendency for the H subunits to be more abundant. For example, in humans, the H subunit is more abundant than the L subunit in 57/77 pairs ( P =3 × 10 −5 , binomial test). Thus, the abundance measurements strongly suggest that a large fraction of complexes will also have uneven stoichiometry within the cell. This trend is consistent across all the organisms considered, including metazoans, yeast and bacteria. The imperfect correspondence between structural stoichiometry and intracellular abundance is not surprising. Many complexes are only transiently formed, particularly those involved in regulatory processes, and might vary widely in concentration over time [37] , [38] . Moreover, some proteins might participate in multiple complexes [39] , [40] . Supplementary Fig. 2 shows the ratios of abundance measurements for subunit pairs with 2:1 stoichiometry. We observe very broad distributions, with many pairs deviating substantially from the 2:1 ratio, yet a clear trend remains for the H subunits to be more abundant. Structural mechanisms for uneven stoichiometry As discussed earlier, in any protein complex with uneven stoichiometry, the H subunits will inherently have some degree of asymmetry and form different interactions within the complex. Here we seek to identify and classify the structural features that facilitate the symmetry breaking necessary for this uneven stoichiometry. For simplicity, we have considered only the 88 non-redundant crystal structures with 2:1 stoichiometry, constituting nearly half of the uneven stoichiometry complexes in our data set ( Fig. 2b ). These complexes are formed from two copies of the H subunit and a single L subunit. Limiting ourselves to 2:1 complexes makes the structural analysis much easier, allowing us to automatically quantify symmetry, conformational changes and binding-site similarity between repeated H subunits, as well as build in extra L subunits and identify steric clashes. The structural determinants in complexes with higher-order uneven stoichiometries are likely to be similar. Through a combination of semi-automated and manual structural analysis, we identified six different mechanisms for facilitating uneven stoichiometry ( Fig. 4 ). 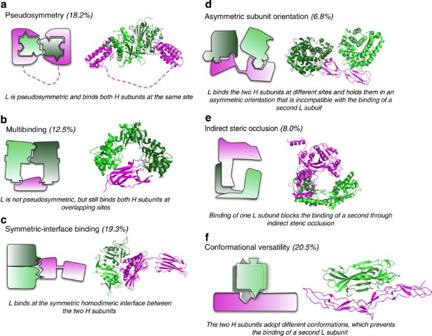Figure 4: Six mechanisms by which protein complexes can achieve uneven stoichiometry. (a) Pseudosymmetry (PDB ID: 3ISM). (b) Multibinding (PDB ID: 1JZD). (c) Symmetric-interface binding (PDB ID: 1HYR). (d) Asymmetric subunit orientation (PDB ID: 2XQW). (e) Indirect steric occlusion (PDB ID: 3Q66). (f) Conformational versatility (PDB ID: 1SG1). Figure 4: Six mechanisms by which protein complexes can achieve uneven stoichiometry. ( a ) Pseudosymmetry (PDB ID: 3ISM). ( b ) Multibinding (PDB ID: 1JZD). ( c ) Symmetric-interface binding (PDB ID: 1HYR). ( d ) Asymmetric subunit orientation (PDB ID: 2XQW). ( e ) Indirect steric occlusion (PDB ID: 3Q66). ( f ) Conformational versatility (PDB ID: 1SG1). Full size image Pseudosymmetry . Although individual polypeptides are not symmetric, they can possess varying degrees of pseudosymmetry. For example, a single protein can have multiple repeats of the same type of domain or can have multiple copies of similar short motifs. If this pseudosymmetry results in multiple copies of the same binding site, this provides a simple mechanism for uneven stoichiometry. In other words, if the L subunit has multiple similar binding sites that allow it to bind multiple H subunits simultaneously, then this pseudosymmetric complex will have uneven stoichiometry. We find that 16/88 (18.2%) 2:1 complexes can be explained by pseudosymmetry. As an example, Fig. 4a shows two molecules of the Drosophila nuclease EndoG in complex with the inhibitor EndoGI [41] . EndoGI consists of repeated domains separated by a disordered linker that allows them to wrap around both sides of the EndoG homodimer, binding each EndoG subunit in a very similar manner. Thus, the pseudosymmetry present in EndoGI allows a single molecule to inhibit both catalytic sites present on opposite sides of the EndoG homodimer. Multibinding . In some cases there is no obvious pseudosymmetry at the level of individual protein chains, yet the same surface on each H subunit is able to interact with different regions on the L subunit. This mechanism is essentially the same as pseudosymmetry, except the H subunits have a multibinding capability: they are able to interact with multiple distinct surfaces through a single region on their own surface. We found that 11/88 (12.5%) cases could be explained by such asymmetric multibinding. Figure 4b shows the 2:1 complex of the Escherichia coli disulphide bond isomerase with the N-terminal domain of the transmembrane electron transporter DsbD [42] . Here, a single DsbD chain is able to use two dissimilar surfaces to bind very similar regions containing the active site on each DsbC molecule. It has been suggested that this asymmetric binding allows DsbD to distinguish oxidized from reduced DsbC [42] . Symmetric-interface binding . There are a number of 2:1 complexes where the L subunit binds directly at the symmetric homodimer interface formed between the two H subunits. Thus, the interaction with L involves only a single binding surface, yet it utilizes the same regions on both H molecules. Although in principle the interacting region of L could have some pseudosymmetry, there are no obvious examples of this in our data set—the binding of L with respect to the two different H subunits is generally asymmetric. This mechanism for facilitating uneven stoichiometry occurs in 17/88 (19.3%) complexes. We illustrate this in Fig. 4c , showing how the homodimeric human-activating immunoreceptor NKG2D binds a single MHC class I-like ligand MICA through its symmetric interface [43] . Here, the edge of the symmetric interface formed between the two NKG2D molecules comprising the receptor is utilized as a binding cleft for the protein ligand. Asymmetric subunit orientation . In the three above scenarios, the single L subunit interacts with similar regions on each H subunit. For these, uneven stoichiometry is very simple to explain, since the binding site is occupied on each H subunit, preventing the binding of a second L subunit. However, in many complexes, the L subunit binds to only a single H subunit, or interacts with completely different regions on each H subunit. In these cases, what prevents a second L subunit from binding and thus forming a complex with even stoichiometry? One possible way to constrain uneven stoichiometry is for the two H subunits to be oriented so that they are asymmetric with respect to each other. If an L subunit binds to both H subunits at different regions, then a twofold axis of rotational symmetry between the H subunits is required to preserve the relative orientation of the two binding surfaces on the other side of the complex. If there is no twofold symmetry, then binding of a second L subunit to both H subunits simultaneously will be blocked. This type of asymmetric intersubunit orientation between the H subunits occurs in 6/88 (6.8%) complexes in our data set. We illustrate this with human factor H in complex with complement C3d [44] ( Fig. 4d ), where factor H binds two copies of C3d at different sites, holding them in an asymmetric orientation. Thus, there are two potential binding surfaces on each C3d, yet only one is occupied. Only a single factor H subunit is able to bind because the relative orientation of the two C3d chains does not permit binding of a second factor H to both. From inspection, this example looks similar to pseudosymmetry ( Fig. 4a ), although the linker between the repeated domains is much shorter. However, although the L subunit in Fig. 4d contains two homologous domains, they bind different surfaces on each H subunit, so binding is not pseudosymmetric. Furthermore, there is no significant difference between the lengths of L subunits from pseudosymmetric and asymmetric subunit orientation complexes, nor between any of the other groups, excluding indirect steric occlusion, discussed below ( Supplementary Fig. 3 ). Thus, chain length does not appear to influence our classifications. Indirect steric occlusion . Uneven stoichiometry can also occur through indirect steric effects. In these cases, a binding site remains open yet, due to indirect steric occlusion, there is not enough physical room to position the full L chain in the correct orientation for binding. Such indirect steric effects explain the 2:1 stoichiometry of 7/88 (8.0%) complexes. Figure 4e shows the example of the Saccharomyces cerevisiae histone chaperone Vps75 in complexes with two molecules of the histone acetyltransferase Rtt109 (ref. 45 ). In this complex, the two Vps75 molecules form a symmetric homodimer through a long helix, while Rtt109 binds primarily to one side of the homodimer. Thus, while the second set of interaction surfaces remains open, the binding of the first large Rtt109 subunit indirectly blocks the binding of the second. Interestingly, we find that although the L subunits of 2:1 complexes generally tend to be smaller than the H subunits, those due to indirect steric occlusion tend to be larger ( Supplementary Fig. 3 ). This suggests that larger L subunits make it less likely that there will physically be room for a second L subunit to bind. Conformational versatility . The fact that different polypeptide chains have identical sequences does not necessarily mean they will adopt identical structures within a complex. Conformational differences between H subunits provide a simple mechanism for uneven stoichiometry by breaking the symmetry between the H subunits and preventing a second L subunit from binding. We find that such conformational versatility can potentially explain uneven stoichiometry in 18/88 (20.5%) complexes. These are complexes where the uneven stoichiometry could not be rationalized by any of the above mechanisms, but moderate-to-large conformational differences are observed between the H subunits. Figure 4f shows the 2:1 complex of human nerve growth factor (NGF) and the receptor p75 (ref. 46 ). As noted in the original publication, binding of p75 induces conformational changes across the NGF homodimer that block the binding of a second p75 subunit. It was suggested that this asymmetric mode of interaction is important for regulation of signalling, as it prevents p75 activation by NGF when p75 is in its dimeric state, with activation only occurring after p75 disassembles into a monomer [46] . Although we classified ~20% of the complexes as having uneven stoichiometry that could likely be explained by conformational versatility, complexes from some other categories also show large conformational differences between repeated H subunits ( Supplementary Fig. 4 ). In particular, the pseudosymmetric and multibinding complexes tend to exhibit large conformational variance. A likely explanation is that in both of these groups, the same surface on both H subunits interacts with different surfaces on L. Differences in the binding of each subunit likely induce different conformational changes. For 13/88 (14.8%) complexes, no structural basis for uneven stoichiometry could be ascertained. For these, a second L subunit with identical interactions to the first could be modelled with no steric clashes ( Supplementary Fig. 5 ). This suggests that the uneven stoichiometry of these complexes might be erroneous. To test this, we manually assigned the stoichiometry of as many of the complexes in our data set as possible by consulting the original publications, in a manner similar to the PiQSi database [47] . Strikingly, we find that in 8/11 complexes where the stoichiometry could be determined from manual inspection of the literature, the quaternary structure of the PDB biological unit was incorrect ( Fig. 5 ). This is highly significant in comparison with all the other groups, where only 5/66 had quaternary structure errors ( P =8 × 10 −6 , Fisher’s exact test). This observation could be useful for assessing the likelihood of a correct quaternary structure assignment: complexes with small conformational differences between repeated subunits, into which stoichiometry-evening subunits can easily be built, are unlikely to truly have uneven stoichiometry. 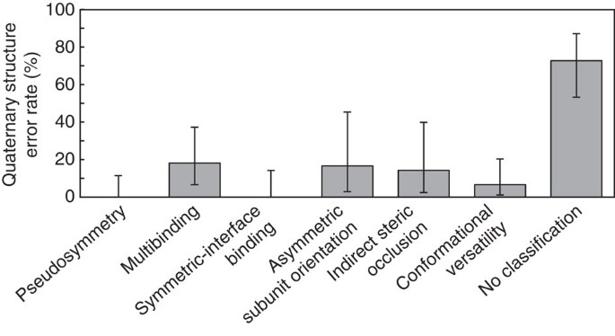Figure 5: Quaternary structure error rates for complexes with uneven stoichiometry from each category. Quaternary structure error rates represent the percentage of complexes for which the quaternary structure in solution as reported in the literature is not consistent with the PDB biological unit. Error bars represent 68% Clopper-Peason binomial confidence intervals. Figure 5: Quaternary structure error rates for complexes with uneven stoichiometry from each category. Quaternary structure error rates represent the percentage of complexes for which the quaternary structure in solution as reported in the literature is not consistent with the PDB biological unit. Error bars represent 68% Clopper-Peason binomial confidence intervals. Full size image Subunit flexibility facilitates uneven stoichiometry Our results suggest that conformational versatility is important for the assembly of many complexes with uneven stoichiometry. A major determinant of the extent to which proteins can change conformation is their intrinsic flexibility: in general, proteins that are more flexible will undergo larger conformational changes on assembly into a complex [48] , [49] , [50] . Therefore, we next investigated what role subunit flexibility might have in facilitating uneven stoichiometry. First, we compared the intrinsic flexibility of subunits from heteromeric complexes with even and uneven stoichiometry using the relative solvent accessible surface area ( A rel ) of their subunits. A rel is a simple parameter that has been shown to be a highly effective proxy for the intrinsic flexibility of both free proteins and the bound subunits of protein complexes [30] , [49] , [50] , [51] , [52] . Interestingly, there is a strong tendency for both H and L subunits of uneven stoichiometry complexes to be more flexible than the subunits of complexes with even stoichiometry ( Fig. 6a ). While this makes sense for H subunits, which often must undergo significant conformational changes to facilitate their varying interactions, this does not explain the increased flexibility of L subunits. In fact, there is a slight tendency for L subunits to be more flexible than the H subunits ( P =0.04, paired Wilcoxon test). 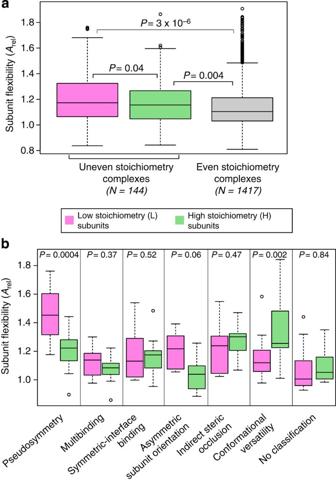Figure 6: The role of subunit flexibility in facilitating uneven stoichiometry. (a) Box plot comparison of subunit flexibility, as measured byArel, for subunits from heteromers with uneven and even stoichiometry. Subunits from complexes with uneven stoichiometry are divided into high (H) and low (L) stoichiometry. Only heteromers with two unique subunit types are considered, due to the strong relationship between subunit flexibility and subunit types per complex30. (b) Box plot comparison of subunit flexibility between H and L subunits from uneven stoichiometry complexes of different classes.Pvalues are calculated with paired (comparisons between H and L subunits) and unpaired (comparisons with even stoichiometry subunits) Wilcoxon tests. Boxes and whiskers indicate the quartile distributions and circles represent outliers. Figure 6: The role of subunit flexibility in facilitating uneven stoichiometry. ( a ) Box plot comparison of subunit flexibility, as measured by A rel , for subunits from heteromers with uneven and even stoichiometry. Subunits from complexes with uneven stoichiometry are divided into high (H) and low (L) stoichiometry. Only heteromers with two unique subunit types are considered, due to the strong relationship between subunit flexibility and subunit types per complex [30] . ( b ) Box plot comparison of subunit flexibility between H and L subunits from uneven stoichiometry complexes of different classes. P values are calculated with paired (comparisons between H and L subunits) and unpaired (comparisons with even stoichiometry subunits) Wilcoxon tests. Boxes and whiskers indicate the quartile distributions and circles represent outliers. Full size image Next, we compared the flexibility of H and L subunits from the different classes of 2:1 complexes identified earlier ( Fig. 6b ). We observe some striking differences between the groups. Most notably, there is a very strong propensity for the L subunits of pseudosymmetric complexes to be more flexible than the H subunits. This can largely be explained by the fact that several of the pseudosymmetric L subunits have two similar domains separated by a long, extended linker that is sometimes disordered, as in the example in Fig. 4a . We might expect this feature also to be common in multibinding, which also involves two sites on the L subunit binding the same regions on the two H subunits. There is a slight but not quite significant tendency for L subunits to be more flexible in multibinding complexes. There is also a strong trend for H subunits to be more flexible than L subunits in conformationally versatile complexes, consistent with the strong association between flexibility and conformational changes on binding. Thus, intrinsic subunit flexibility appears to be important for facilitating the varying conformations required by sequence-identical subunits to form different interactions. It is interesting to consider these results in light of our recent work showing that more flexible subunits of heteromeric complexes tend to have been acquired more recently in evolution [30] . If this trend is followed in the present data set of 2:1 complexes (as it was for nearly 80% of human heteromers previously investigated), it would suggest that overall there is a slight tendency for H subunits to evolve before L subunits, particularly in the pseudosymmetry and asymmetric subunit orientation groups. However, for the conformational versatility group, the more flexible subunits may tend to have evolved after the more rigid L subunits. A much larger data set of uneven stoichiometry complexes would be required to test this directly. Uneven stoichiometry across evolution The way quaternary structure space is populated varies substantially across evolutionarily diverse organisms. For example, eukaryotes generally have a higher proportion of heteromers than prokaryotes [30] , [53] . Furthermore, eukaryotic heteromers tend to contain more distinct subunit types, which is partially facilitated by the increased flexibility of eukaryotic proteins [30] . Therefore, given that both an increased number of subunit types and increased flexibility are associated with uneven stoichiometry, we might also expect that the fraction of complexes with uneven stoichiometry should be enriched in eukaryotes. In Fig. 7a , we compare the percentages of heteromeric crystal structures with uneven stoichiometry in different evolutionary groups. Surprisingly, bacteria are significantly enriched in complexes with uneven stoichiometry compared with eukaryotes (15.0 versus 8.3%, P =0.0002, Fisher’s exact test). Archaea are similar to eukaryotes (8.5%) and viruses are intermediate (12.0%), although there are far fewer heteromers from these groups and the differences are not statistically significant. Bacteria also have a higher proportion of heteromers with uneven stoichiometry in the NMR, EM and IntAct data sets, although only statistically significant for IntAct ( Supplementary Fig. 6 ). 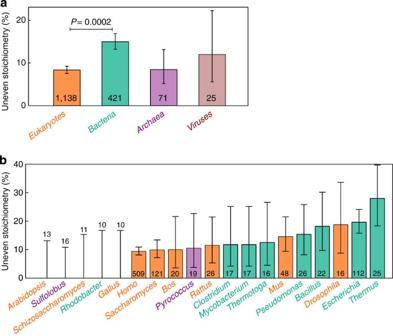Figure 7: Evolutionary prevalence of heteromeric complexes with uneven stoichiometry. Fraction of heteromeric crystal structures with uneven stoichiometry from the different domains of life and viruses (a), and from those genera having at least 10 structures in our non-redundant data set (b). The difference between eukaryotes and bacteria is highly significant (Fisher’s exact test), but the differences between other domains are not (due to the vastly smaller sample sizes). The numbers of heteromers in each evolutionary group are shown. Error bars represent 68% Clopper–Pearson binomial confidence intervals. Figure 7: Evolutionary prevalence of heteromeric complexes with uneven stoichiometry. Fraction of heteromeric crystal structures with uneven stoichiometry from the different domains of life and viruses ( a ), and from those genera having at least 10 structures in our non-redundant data set ( b ). The difference between eukaryotes and bacteria is highly significant (Fisher’s exact test), but the differences between other domains are not (due to the vastly smaller sample sizes). The numbers of heteromers in each evolutionary group are shown. Error bars represent 68% Clopper–Pearson binomial confidence intervals. Full size image In Fig. 7b , we break down the comparison by genera. A clear difference between bacteria and eukaroyotes is still observed. For example, 7 of the 9 genera with the highest proportions of uneven stoichiometry are bacterial, whereas 7 of the 10 with the lowest proportions are eukaryotic. Thermus has the highest proportion of uneven stoichiometry (28.0%), followed by Escherichia (19.6%). Although Drosophila has a relatively high proportion of uneven stoichiometry (18.8%), this comes from only 3/16 heteromers, so the confidence interval is much larger. In humans, the largest group, only 48/509 (9.4%), have uneven stoichiometry. Overall, these results strongly suggest an evolutionary enrichment of uneven stoichiometry in bacterial heteromers. This is despite the increased flexibility of eukaryotic proteins and the tendency for eukaryotic complexes to have more distinct subunit types [30] , both factors that appear to promote uneven stoichiometry. How can we explain this? Since eukaryotic proteins tend to be longer than those from bacteria [54] , this could explain our observation if shorter subunits are associated with an increased propensity for uneven stoichiometry. However, we observe no significant length difference between the subunits of even and uneven stoichiometry complexes ( Supplementary Fig. 7 ), suggesting that protein length is not an important determinant of uneven stoichiometry. Another possible explanation is related to the well-known observation that many eukaryotic heteromers have paralogous subunits that presumably evolved via ancestral gene duplication events [55] . Thus, one could imagine that in some eukaryotic homologues of bacterial complexes with uneven stoichiometry, the higher stoichiometry subunits in bacteria could now be paralogues. For example, a 2:1 complex might have evolved into a 1:1:1 complex through a duplication of the gene encoding the H subunit. To test this, in Supplementary Fig. 8 we consider stoichiometry not at the level of distinct subunits, but instead at the level of PFAM [56] domain architecture, so that paralogues will be treated as identical. A significant increase in uneven stoichiometry in bacteria is conserved across different experimental methods, strongly suggesting that gene duplication cannot explain these results. Evolutionary variation in self-assembly propensity As heteromers with uneven stoichiometry all have at least one repeated subunit, we wondered whether there might be differences in the self-assembly propensities of bacterial and eukaryotic proteins. That is, are bacterial proteins more likely to form homomeric interactions with other copies of themselves, and could this explain their increased uneven stoichiometry? 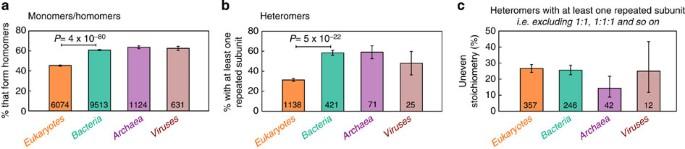Figure 8: Variation in self-assembly propensities across evolution. (a) Percentage of non-redundant crystal structures involving just a single polypeptide chain that self-assemble to form homomeric complexes, with the rest remaining monomeric. (b) Percentage of heteromeric crystal structures where at least one of the subunits is repeated within the complex. (c) Percentage of heteromers with uneven stoichiometry when complexes without subunit repeats (e.g., with 1:1 or 1:1:1 stoichiometry) are excluded.Pvalues are calculated with Fisher’s exact test. Error bars represent 68% Clopper–Pearson binomial confidence intervals. Figure 8a compares the percentage of individual polypeptide chains that can self-assemble to form homomers across different evolutionary groups. Interestingly, eukaryotic proteins are the least likely to form homomers. In fact, most individual eukaryotic proteins are monomeric, whereas most bacterial, archaeal and viral proteins are homomeric. A similar analysis, split into individual genera, is shown in Supplementary Fig. 9 . Figure 8: Variation in self-assembly propensities across evolution. ( a ) Percentage of non-redundant crystal structures involving just a single polypeptide chain that self-assemble to form homomeric complexes, with the rest remaining monomeric. ( b ) Percentage of heteromeric crystal structures where at least one of the subunits is repeated within the complex. ( c ) Percentage of heteromers with uneven stoichiometry when complexes without subunit repeats (e.g., with 1:1 or 1:1:1 stoichiometry) are excluded. P values are calculated with Fisher’s exact test. Error bars represent 68% Clopper–Pearson binomial confidence intervals. Full size image Next, we performed an analogous comparison for heteromers. Figure 8b shows the percentage of heteromers that have at least one repeated subunit (that is, they do not have 1:1, 1:1:1, etc . stoichiometry). The results are similar to homomers, with most eukaryotic heteromers having no subunit repeats, and most heteromers from other groups having repeats. In Supplementary Fig. 10 , we show that neither these results, nor those in Fig. 7a , are due to the fact that many eukaryotic crystal structures are fragments of full-length proteins (for example, individual domains), as they are robust when only close-to-full-length proteins are considered. Figure 8a,b reveals that the propensity for protein self-assembly is much higher in bacteria than eukaryotes. To test whether this could explain the increased uneven stoichiometry in bacteria, in Fig. 8c we plot the percentage of heteromers with uneven stoichiometry, excluding those with no subunits repeats. Here, bacteria and eukaryotes are nearly identical. Thus, it appears that the evolutionary differences in uneven stoichiometry can be largely explained by differences in self-assembly propensities, which is also reflected in the much lower tendency for eukaryotic proteins to assemble into homomeric complexes or into heteromers with subunit repeats. There is another prediction we can make from this. Many heteromers with uneven stoichiometry are partially formed via homomeric self-assembly, in which one subunit interacts with another copy of itself. However, some complexes (for example, Fig. 4d ), involve only heteromeric interactions. If the increased uneven stoichiometry in bacteria is really due to an increased propensity for self-assembly, then we should expect this to be driven by complexes that form homomeric interactions between the higher stoichiometry subunits. Conversely, we do not expect a significant difference between bacteria and eukaryotes in the proportion of complexes with uneven stoichiometry formed only by heteromeric interactions. The data confirm this: specifically, only 57/95 (60.0%) of eukaryotic complexes with uneven stoichiometry are formed via homomeric interactions, compared with 57/63 (90.5%) of those from bacteria ( P =2 × 10 −5 , Fisher’s exact test) ( Supplementary Fig. 11 ). Furthermore, increased uneven stoichiometry of bacteria is no longer present when only complexes with no homomeric interactions are considered. This strongly suggests that the enrichment in bacterial complexes with uneven stoichiometry is linked to a general increase in the propensity for homomeric interactions in bacteria versus eukaryotes. Understanding protein quaternary structure is important for understanding protein function. With the ability of large-scale proteomic experiments to characterize the components and stoichiometries of protein complexes, there is a need to put these results in a structural context. Elucidating the fundamental principles that determine quaternary structure topologies is crucial to this. In combination with homology modelling, we will eventually be able to obtain much more complete structural representations of in vivo interactomes. Here we have made important steps in our understanding of protein complexes with uneven stoichiometry, which comprise ~10% of heteromeric complexes in vitro , and probably a much greater percentage in vivo , given the likelihood that intracellular complexes tend to have more distinct subunits [30] , [31] . To understand the structural determinants of uneven stoichiometry, we focused primarily on the most prevalent group: those with 2:1 stoichiometry. This made a systematic analysis far more feasible. In principle, the origins of complexes with higher-order uneven stoichiometries should be quite similar. This is especially so for those complexes with the same 2:1 reduced subunit ratio, which comprise the majority of the remaining complexes. These can be formed simply through symmetric repetition of the 2:1 unit (for example, 4:2 or 6:3) or addition of new chains interacting stoichiometrically with the H or L subunits (for example, 2:2:1 or 2:1:1). In addition, the fact that 2:1 ratios are by far the most common uneven stoichiometry could be useful for prioritizing quaternary structure search space in protein complex modelling. The six categories of uneven stoichiometry we identified have some potential overlap. For instance, the difference between pseudosymmetry and multibinding depends on a somewhat qualitative assessment of the presence of pseudosymmetry. In fact, we can probably consider the differences between pseudosymmetry and multibinding as a continuum, ranging from perfect domain repeats, to degenerate binding motifs, to structurally similar binding sites that lack any sequence similarity, to clearly different binding regions that are able to interact with overlapping surfaces. Similarly, symmetric-interface binding could be considered a special case of multibinding where a single binding surface on L interacts with the same position on both H molecules. Finally, the amount of conformational change needed to block the binding of a second L chain will vary from case to case, so in some cases we can only speculate that uneven stoichiometry is due to conformational versatility. Here we showed that evolutionary variations in uneven stoichiometry can be explained by differences in self-assembly propensity. However, the origins of the evolutionary differences in self-assembly propensity are still unclear. One hypothesis is that this could reflect fundamentally different utilizations of quaternary structure space by prokaryotes and eukaryotes due to markedly different proteome size. Given that bacteria tend to have smaller genomes encoding fewer proteins, it may be that they have taken greater advantage of uneven stoichiometry and self-assembly as a strategy of coding economy, to evolve more different quaternary structure topologies from fewer protein-coding genes. In other words, bacteria are utilizing a larger region of the available quaternary structure space. In contrast, eukaryotes have more proteins available with which to construct their complexes. However, we do note that both Saccharomyces and archaeal species have relatively small genomes and also low propensities for uneven stoichiometry and self-assembly. Thus, it may not be genome size itself that is responsible for the phenomena, but instead could be reflective of some other fundamental difference between prokaryotes and eukaryotes. For example, perhaps homomeric interactions are less energetically favourable in eukaryotes, for example, due to their much larger cell size, and thus there has been less evolutionary selection for protein self-assembly. Determining the structures of more protein complexes from more evolutionarily diverse organisms will be helpful for addressing this issue conclusively. Protein complex data sets The data set of heteromeric crystal structures used here was taken from the PDB on 2012-08-08 and is very similar to that used in a recent study [30] . The main difference is that complexes known to have quaternary structure assignment errors are not excluded here, as we utilized these for the analysis of quaternary structure error rates in different groups. Redundancy filtering was performed at the level of 50% sequence identity and subunit stoichiometry—if two complexes share the same stoichiometry, with all subunits sharing >50% sequence identity, only one complex was considered in our non-redundant data set. Furthermore, we manually obtained quaternary structure assignments for most of the heteromers with uneven stoichiometry used in this study, very similar to what was done with the PiQSi database [47] . The full set of heteromeric crystal structures used in this study is provided in Supplementary Data 1 . IntAct complexes and NMR and EM structures from the PDB were also filtered for redundancy at the 50% sequence identity level. Any IntAct complexes with cross references to PDB structures were excluded. The non-redundant heteromers from these data sets are provided in Supplementary Data 2 . Classification of uneven stoichiometry To classify the 2:1 stoichiometry complexes, we employed a semi-automated approach. First, we automatically identified those complexes where a single L subunit binds the two H subunits at the same position on each H. Through manual inspection of each structure, we classified these as follows: pseudosymmetry, if the L subunit contained repeated domains or shorter motifs that facilitated the similar binding to each H subunit; multibinding, if there was no obvious pseudosymmetry; and symmetric-interface binding, if the L subunit binds at the homodimeric interface between the two H subunits. Next, we considered those remaining complexes where the L subunit does not directly occlude the same binding surface on each H subunit. We calculated the angle of rotation between each pair of H subunits using lsqkab [57] , [58] to identify those that deviate from twofold rotational symmetry; these were classified as asymmetric subunit orientation . For the remaining complexes, we then attempted to build in a second L subunit by considering the alignment of the existing L subunit with respect to one of the H subunits, and then adding a new L subunit with the same relative orientation with respect to the other H subunit. We then automatically identified those 2:2 complexes that contained steric clashes involving the new L subunit; these were classified as indirect steric occlusion. Classification of complexes into the above categories is highly objective (barring the qualitative aspect of distinguishing pseudosymmetry from multibinding), and it is simple to physically understand why these complexes could not have even stoichiometry. However, for the final category, conformational versatility, it is difficult to know exactly the extent of conformational changes required for uneven stoichiometry. We set a threshold of >1.6 Å all-atom root mean squared deviation (r.m.s.d. ), which maximized the segregation between complexes with and without quaternary structure errors in the ‘no classification’ and ‘conformational versatility’ categories. We also classified one complex close to the threshold (PDB ID: 3EJJ) as ‘conformational versatility’ because the original paper described the uneven stoichiometry as arising due to structural changes near the binding site [59] . In Supplementary Fig. 12 , we show that, even independent of our categorization of complexes as ‘conformational versatility’ versus ‘no classification’, there is still a very strong tendency for complexes with quaternary structure assignment errors to have small r.m.s.d. values. Comparison of protein abundance and stoichiometry For the protein abundance analysis, we mapped all the subunits from heteromeric crystal structures with uneven stoichiometry (prior to sequence redundancy filtering) against the sequences of proteins from different organisms present in PaxDB [35] , and Proteome DB [36] for humans. Considering each organism separately, for each pair of H and L subunits we identified the pair of proteins having abundance measurements and sharing the highest sequence identity (minimum 70%) to the protein complex chains. A given pair of proteins was only associated with a single pair of H and L subunits in our data set. For species with multiple PaxDB data sets, we used the ‘whole organism integrated’ data sets. All H and L subunits with corresponding abundance measurements from each species are provided in Supplementary Data 4 . How to cite this article: Marsh, J. A. et al . Structural and evolutionary versatility in protein complexes with uneven stoichiometry. Nat. Commun . 6:6394 doi: 10.1038/ncomms7394 (2015).